ABCA4 is anN-retinylidene-phosphatidylethanolamine and phosphatidylethanolamine importer ATP-binding cassette (ABC) transporters comprise a superfamily of proteins, which actively transport a variety of compounds across cell membranes. Mammalian and most eukaryotic ABC transporters function as exporters, flipping or extruding substrates from the cytoplasmic to the extracellular or lumen side of cell membranes. Prokaryotic ABC transporters function either as exporters or importers. Here we show that ABCA4, an ABC transporter found in retinal photoreceptor cells and associated with Stargardt macular degeneration, is a novel importer that actively flips N -retinylidene-phosphatidylethanolamine from the lumen to the cytoplasmic leaflet of disc membranes, thereby facilitating the removal of potentially toxic retinoid compounds from photoreceptors. ABCA4 also actively transports phosphatidylethanolamine in the same direction. Mutations known to cause Stargardt disease decrease N -retinylidene-phosphatidylethanolamine and phosphatidylethanolamine transport activity of ABCA4. These studies provide the first direct evidence for a mammalian ABC transporter that functions as an importer and provide insight into mechanisms underlying substrate transport and the molecular basis of Stargardt disease. ATP-binding cassette (ABC) transporters comprise a superfamily of membrane proteins widely distributed in all prokaryotic and eukaryotic organisms [1] , [2] , [3] . ABC transporters typically utilize the energy from ATP binding and hydrolysis to transport chemically diverse substrates across biological membranes, including nutrients, drugs, antibiotics, vitamins, lipids, amino acids, inorganic ions, polypeptides and polysaccharides. The importance of ABC transporters is highlighted by the finding that many are linked to severe genetic diseases [4] . At a structural level, ABC transporters consist of two transmembrane domains with multiple membrane-spanning segments and two cytoplasmic nucleotide-binding domains (NBDs), each containing a Walker A and B motif and a signature C motif characteristic of ABC proteins. The four domains can reside within a single polypeptide known as a full transporter or in two or more different polypeptides, which associate to form a functional complex. Prokaryotic ABC transporters are known to function either as importers or exporters [5] , [6] . Most well-characterized eukaryotic ABC transporters, however, have been shown to function as exporters transporting substrates from the cytoplasmic to the exocytoplasmic (extracellular or lumen) side of biological membranes. This has led many investigators to propose that all eukaryotic ABC transporters have evolved to be exporters [1] , [7] . High-resolution structures have yielded a generalized model in which ABC importers and exporters alternate between inward and outward substrate accessible conformations depending on the binding of ATP to the its NBDs [1] , [5] , [6] , [7] . Mammalian ABC proteins have been divided into seven subfamilies (ABCA through ABCG) based on similarities in gene organization and sequence [8] . The ABCA subfamily consists of 12 members and has attracted considerable attention in recent years since genetic defects in several members have been linked to severe human diseases [9] . Mutations in ABCA1 cause Tangier disease, a disorder associated with the accumulation of cholesterol in peripheral tissues and a decrease in circulating HDL [10] . ABCA3 mutations cause neonatal surfactant deficiency, a disease linked to the loss in surfactant lipid secretion from alveolar type II lung cells [11] . Defects in ABCA12 are responsible for harlequin ichthyosis, a skin disorder caused by defective lipid transport [12] . Although cell-based studies have indicated that many ABCA transporters are involved in lipid transport, the identity of their substrates and direction of transport have not been defined at a biochemical level. ABCA4, also known as ABCR or the rim protein, is another key member of the ABCA subfamily linked to genetic diseases [13] . Over 800 mutations in the ABCA4 gene are now known to cause Stargardt macular degeneration, a relatively common early onset recessive disease characterized by the loss in central vision, progressive bilateral atrophy of photoreceptor and retinal pigment epithelial cells, accumulation of fluorescent deposits in the macula, and a delay in dark adaptation [14] , [15] . Mutations in ABCA4 are also responsible for other severe retinal degenerative diseases, including cone-rod dystrophy, retinitis pigmentosa and age-related macular degeneration [16] , [17] . ABCA4 is a full transporter organized in two tandem-arranged halves, each consisting of a membrane-spanning segment, followed by a large exocytoplasmic domain, a transmembrane domain and a cytoplasmic NBD [18] , [19] . Missense mutations, the largest class of mutations associated with Stargardt disease, are distributed throughout the 2273 amino-acid polypeptide chain. Several studies have suggested that ABCA4 functions as a retinoid transporter facilitating the clearance of potentially toxic all- trans retinal (ATR) from photoreceptors following photoexcitation. ABCA4 is localized with opsin photopigments in outer segment disc membranes of rod and cone photoreceptor cells [18] , [20] , [21] . Purified ABCA4 reconstituted into phosphatidylethanolamine (PE)-containing lipid vesicles displays a basal ATPase activity, which is stimulated two- to fivefold by all- trans or 11- cis retinal [22] , [23] . N -retinylidene-PE, the Schiff base adduct of retinal and PE, binds with high affinity to purified ABCA4 and is released by ATP suggesting that this compound may be the physiological substrate for ABCA4 [24] . Abca4 knockout mice display a light-dependent accumulation of ATR, PE and N -retinylidene-PE in retina tissue, progressive buildup of lipofuscin and the di-retinal-pyridinium-ethanolamine compound A2E in retinal pigment epithelial cells, and a delay in dark adaptation consistent with decreased clearance of ATR from disc membranes [25] , [26] . Taken together these studies have led to a model in which ABCA4 functions as an active transporter, which flips N -retinylidene-PE across photoreceptor disc membranes thereby enabling ATR to be reduced to all- trans retinol by the cytoplasmic retinol dehydrogenase RDH8 following the dissociation of N -retinylidene-PE into retinal and PE [23] , [25] , [27] . Although there is support for the role of ABCA4 in the removal of retinoids from disc membranes, direct biochemical evidence for the function of ABCA4 as a retinoid transporter is lacking. Furthermore, the proposed 'import' direction of transport from the lumen to cytoplasmic side of the disc membrane is counter to the 'export' direction proposed for all other mammalian ABC transporters. This has raised the following questions: does ABCA4 really transport retinal or N -retinylidene-PE? Are all mammalian ABC proteins exporters or are some such as ABCA4 importers? What is mechanism of substrate transport by ABCA4? What is the effect of disease-causing mutations on the transport activity of ABCA4? The development of biochemical assays, which can directly measure retinoid transport and resolve some of these issues has been impeded by the hydrophobic nature of retinoid compounds, their rapid diffusion across lipid bilayers and between lipid vesicles [28] , [29] , and the unstable nature of N -retinylidene-PE, for example, N -retinylidene-PE is in equilibrium with retinal and PE [24] . In the present study, we show for the first time that ABCA4 functions as a novel N -retinylidene-PE and PE importer translocating these substrates from the lumen to the cytoplasmic side of photoreceptor disc membranes. We have also analysed the retinoid transport function for a number of ABCA4 mutants providing new insight into the molecular basis for Stargardt disease. ATP-dependent transfer of retinal between lipid vesicles To characterize the transport function of ABCA4, we have developed a biochemical assay that measures ATP-dependent transfer of radiolabelled retinoids from ABCA4-containing donor proteoliposomes to acceptor liposomes. The basis for this assay is illustrated in Fig. 1 . ATR rapidly equilibrates between the two vesicle populations [29] and reversibly reacts with PE to form N -retinylidene-PE, a portion of which is trapped in the inner leaflet of the vesicles. Using ATP as an energy source, ABCA4 transports N -retinylidene-PE from the inner to the outer leaflet of the proteoliposomes. The increase in N -retinylidene-PE on the outer leaflet coupled with its dissociation into ATR and PE results in a net solution transfer of ATR to the acceptor liposomes, where it reacts with PE to form N -retinylidene-PE. 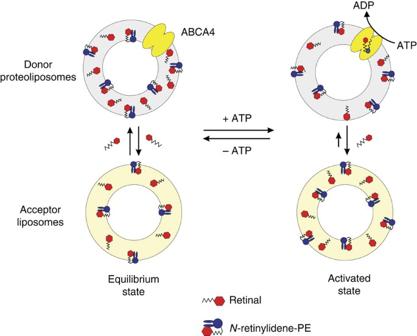Figure 1: Schematic diagram showing the rationale for ABCA4-catalysed retinoid transport activity between donor and acceptor vesicles. In the absence of ATP (equilibrium state), retinal rapidly equilibrates between the donor proteoliposomes (or disc membranes) containing ABCA4 and acceptor liposomes. The distribution of retinal in each population is dependent on their phospholipid composition. Retinal freely diffuses in the lipid bilayer and reacts with PE to form an equilibrium mixture withN-retinylidene-PE, which is distributed on both sides of the lipid bilayer. Free PE is not shown for simplicity. Addition of ATP to the NBDs of ABCA4 results in the active transport or flipping ofN-retinylidene-PE from the lumen side of the bilayer to the outside (equivalent to the cytoplasmic) of the bilayer resulting in an accumulation ofN-retinylidene-PE on the outer leaflet. This increase coupled with its dissociation to PE and retinal results in a higher concentration of retinal on the outer leaflet and a net transfer of retinal to the acceptor liposomes. This can be measured by determining the accumulation of radiolabelled retinoid in the liposome after separation from donor proteoliposomes by centrifugation. The density of the liposomes is increased by encapsulated sucrose thereby facilitating separation by centrifugation. If ATP is removed such as by chelation of Mg2+with EDTA or ABCA4 is inactivated by an inhibitor, retinal flows back to the proteoliposomes to generate an equilibrium state similar to the initial state. Figure 1: Schematic diagram showing the rationale for ABCA4-catalysed retinoid transport activity between donor and acceptor vesicles. In the absence of ATP (equilibrium state), retinal rapidly equilibrates between the donor proteoliposomes (or disc membranes) containing ABCA4 and acceptor liposomes. The distribution of retinal in each population is dependent on their phospholipid composition. Retinal freely diffuses in the lipid bilayer and reacts with PE to form an equilibrium mixture with N -retinylidene-PE, which is distributed on both sides of the lipid bilayer. Free PE is not shown for simplicity. Addition of ATP to the NBDs of ABCA4 results in the active transport or flipping of N -retinylidene-PE from the lumen side of the bilayer to the outside (equivalent to the cytoplasmic) of the bilayer resulting in an accumulation of N -retinylidene-PE on the outer leaflet. This increase coupled with its dissociation to PE and retinal results in a higher concentration of retinal on the outer leaflet and a net transfer of retinal to the acceptor liposomes. This can be measured by determining the accumulation of radiolabelled retinoid in the liposome after separation from donor proteoliposomes by centrifugation. The density of the liposomes is increased by encapsulated sucrose thereby facilitating separation by centrifugation. If ATP is removed such as by chelation of Mg 2+ with EDTA or ABCA4 is inactivated by an inhibitor, retinal flows back to the proteoliposomes to generate an equilibrium state similar to the initial state. Full size image The increase in retinoid in the acceptor liposomes can be quantified after separation from the proteoliposomes. The separation of the dense acceptor vesicles from donor proteoliposomes by centrifugation is highly efficient as analysed using fluorescently labelled lipids ( Supplementary Table S1 ) and occurs without vesicle fusion as confirmed by fluorescent lipid-quenching measurements ( Supplementary Table S2 ). 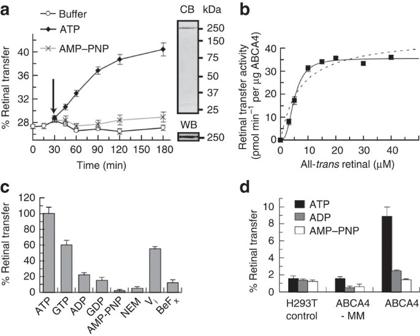Figure 2: ATP-dependent transfer of ATR from donor ABCA4 proteoliposomes to acceptor liposomes. Donor proteoliposomes consisted of DOPC, DOPE and BPL at a weight ratio of 6:2:2 reconstituted with ABCA4 purified from either (a–c) bovine ROS membranes or (d) ABCA4-transfected HEK293 cell extracts. Acceptor liposomes consisted of DOPC and DOPE at a weight ratio of 7:3. (a) Time course for the transfer of [3H] ATR from donor proteoliposomes to acceptor liposome vesicles. [3H] ATR rapidly distributed between donor proteoliposomes and acceptor liposomes with ~28% of the ATR partitioning into the acceptor liposomes at 37 °C. After 30 min, 2 mM ATP or AMP–PNP or control buffer was added (arrow) and radioactivity in the acceptor liposomes was measured at various times. Data are plotted as a mean with error bars representing±s.e.m. forn=3. Coomassie blue (CB)-stained gel and western blot (WB) shows the purity of the ABCA4 used for reconstitution. (b) ATP-dependent rate of [3H] ATR transfer as a function of ATR concentration. Solid line shows best-fit sigmoidal curve forK0.5of 4.9±0.2 μM and aVmaxof 35.5±0.7 pmol min−1per μg protein yielding a Hill coefficient of 2.3±0.3. Dotted line shows a best-fit Michaelis–Menten curve for comparison. (c) The effect of nucleotides (1 mM) and inhibitors (10 mM NEM, 1 mM orthovanadate (Vi) or 0.2 mM beryllium fluoride (BeFx)) on [3H] ATR transfer from proteoliposomes to liposomes. Percent relative retinal transfer activity data displayed as a mean with error bars representing±s.e.m forn=3. (d) Effect of ATP, ADP and AMP–PNP on [3H] ATR transfer from donor proteoliposomes reconstituted with WT ABCA4 or the ATPase-impaired K969M/K1978M double mutant (ABCA4-MM) purified from transfected HEK293 cells. ATR concentration was 10 μM. Data are plotted as a mean with error bars representing±s.e.m forn=3. Figure 2a–c shows the results of experiments using donor proteoliposomes reconstituted with ABCA4 purified from photoreceptor rod outer segments (ROS). [ 3 H]-ATR rapidly partitioned between the donor proteoliposomes and acceptor liposomes with approximately 28% of the retinoid being present in the liposomes ( Fig. 2a ). Addition of 2 mM ATP resulted in a linear increase in transfer of [ 3 H]-ATR from the donor to acceptor vesicles for 60 min. The rate of transfer was dependent on the ATR concentration and showed sigmoidal kinetics with a K 0.5 of 4.9±0.2 μM, a V max of 35.5±0.7 pmol min −1 per μg of protein, and a Hill coefficient of 2.3±0.3 at 37 °C ( Fig. 2b ). ATP-dependent transfer of [ 3 H]-ATR increased with increasing amounts of ABCA4 and was specific for ATR, as ATP-dependent transfer was not observed for [ 3 H]-all- trans retinol ( Supplementary Fig. S1 ). Removal of MgATP by EDTA chelation of Mg 2+ led to a reduction in accumulated ATR in the acceptor liposomes ( Supplementary Fig. S2 ). Figure 2: ATP-dependent transfer of ATR from donor ABCA4 proteoliposomes to acceptor liposomes. Donor proteoliposomes consisted of DOPC, DOPE and BPL at a weight ratio of 6:2:2 reconstituted with ABCA4 purified from either ( a – c ) bovine ROS membranes or ( d ) ABCA4-transfected HEK293 cell extracts. Acceptor liposomes consisted of DOPC and DOPE at a weight ratio of 7:3. ( a ) Time course for the transfer of [ 3 H] ATR from donor proteoliposomes to acceptor liposome vesicles. [ 3 H] ATR rapidly distributed between donor proteoliposomes and acceptor liposomes with ~28% of the ATR partitioning into the acceptor liposomes at 37 °C. After 30 min, 2 mM ATP or AMP–PNP or control buffer was added (arrow) and radioactivity in the acceptor liposomes was measured at various times. Data are plotted as a mean with error bars representing±s.e.m. for n =3. Coomassie blue (CB)-stained gel and western blot (WB) shows the purity of the ABCA4 used for reconstitution. ( b ) ATP-dependent rate of [ 3 H] ATR transfer as a function of ATR concentration. Solid line shows best-fit sigmoidal curve for K 0.5 of 4.9±0.2 μM and a V max of 35.5±0.7 pmol min −1 per μg protein yielding a Hill coefficient of 2.3±0.3. Dotted line shows a best-fit Michaelis–Menten curve for comparison. ( c ) The effect of nucleotides (1 mM) and inhibitors (10 mM NEM, 1 mM orthovanadate (V i ) or 0.2 mM beryllium fluoride (BeF x )) on [ 3 H] ATR transfer from proteoliposomes to liposomes. Percent relative retinal transfer activity data displayed as a mean with error bars representing±s.e.m for n =3. ( d ) Effect of ATP, ADP and AMP–PNP on [ 3 H] ATR transfer from donor proteoliposomes reconstituted with WT ABCA4 or the ATPase-impaired K969M/K1978M double mutant (ABCA4-MM) purified from transfected HEK293 cells. ATR concentration was 10 μM. Data are plotted as a mean with error bars representing±s.e.m for n =3. Full size image The effect of nucleotides and ATPase inhibitors on the rate of [ 3 H]-ATR transfer was investigated. When ATP was replaced with its non-hydrolyzable derivative, AMP–PNP, no significant [ 3 H]-ATR transfer was observed above background implicating ATP hydrolysis in the transfer reaction ( Fig. 2a,c ). GTP could partially substitute for ATP, whereas ADP and GDP showed substantially reduced activity. The sulfhydryl reagent N -ethylmaleimide (NEM) previously shown to inhibit the ATPase activity of ABCA4 [22] , also inhibited [ 3 H]-ATR transfer to acceptor vesicles. Orthovanadate, a phosphate analogue and a weak inhibitor of ABCA4 ATPase activity [23] , partially inhibited the [ 3 H]-ATR transfer at a concentration of 1 mM, whereas 0.2 mM beryllium fluoride, another phosphate analogue, strongly inhibited [ 3 H]-ATR transfer. The effect of various divalent metal ions on the ATR transfer reaction was studied ( Supplementary Fig. S3 ). Transfer activity was observed with either Mg 2+ or Mn 2+ , but not Zn 2+ or Ca 2+ . Although ABCA4 isolated from ROS by immunoaffinity chromatography has been shown to be highly pure [22] , [23] , [30] , it is possible that a residual protein contaminant may be responsible for the ATP-dependent [ 3 H]-ATR transfer. This was examined using donor proteoliposomes reconstituted with wild-type (WT) ABCA4 or the ATPase deficient K969M/K1978M double mutant (ABCA4-MM) ( Fig. 2d ). ATP-dependent [ 3 H]-ATR transfer was observed for WT ABCA4, but not ABCA4-MM. These studies provide strong evidence that ATP-dependent ATR transfer from donor to acceptor vesicles is mediated by ABCA4 and displays many characteristic properties previously observed for retinal-stimulated ATPase activity of ABCA4 [22] , [23] . Non-protonated N -retinylidene-PE is a substrate for ABCA4 To further identify the substrate for ABCA4, we examined the effect of all- trans retinol as an analogue of ATR and N -retinyl-PE as a stabilized reduced derivative of N -retinylidene-PE on the [ 3 H]-ATR transfer reaction. All- trans retinol had no effect on the [ 3 H]-ATR transfer, whereas N -retinyl-PE strongly inhibited the transfer with an IC 50 of 9 μM ( Fig. 3a ). As N -retinylidene-PE is in equilibrium with ATR and PE, the ATP-dependent [ 3 H]-ATR transfer reaction should depend on PE. ATR transfer does not occur when ABCA4 is reconstituted into phosphatidylcholine (PC) vesicles lacking PE ( Fig. 3b ). Furthermore, transfer is strongly dependent on the PE concentration ( Fig. 3c ). 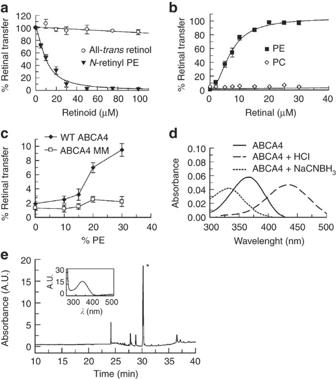Figure 3: Effect of retinoids and PE on ATP-dependent transfer of ATR from donor proteoliposomes to acceptor liposomes. (a) Inhibition of ATP-dependent [3H] ATR transfer (10 μM) from ABCA4-containing donor proteoliposomes to acceptor liposomes with increasing concentrations of all-transretinol orN-retinyl-PE. Donor proteoliposomes were reconstituted with ABCA4 purified from bovine ROS membranes. Percent-relative retinal transfer plotted as a mean with error bars representing±s.d. forn=3. (b) ATP-dependent transfer of [3H] ATR from ABCA4-containing proteoliposomes composed of only DOPC (PC) or DOPC containing 30% DOPE (PE). Sigmoidal curve for PE was generated and yielded aK0.5=6.7 μM±0.3 with a Hill coefficient of 2.1±0.2. Percent relative retinal transfer plotted as a mean with error bars representing±s.d. forn=3. (c) Effect of increasing DOPE on the ATP-dependent transfer of [3H] ATR from DOPC/DOPE proteoliposomes reconstituted with either WT ABCA4 or ABCA4-MM mutant. Data was plotted as mean with error bars representing±s.e.m. forn=6. (d) Absorption spectra of purified ABCA4 with bound retinoid substrate. Spectrum at neutral pH (solid line) shows a maximum of 360 nm characteristic of non-protonatedN-retinylidene-PE. Treatment with HCl resulted in an absorption maximum of 440 nm characteristic of protonatedN-retinylidene-PE. Treatment with NaCNBH3resulted in a shift to 330 nm characteristic ofN-retinyl-PE. (e) HPLC chromatograph of NaCNBH3reduced retinoid substrate in ABCA4 withy-axis in absorbance units (A.U.). Retention time and absorption spectrum (inset) of the predominant peak (*) showing aλ-max at 330 nm. Figure 3: Effect of retinoids and PE on ATP-dependent transfer of ATR from donor proteoliposomes to acceptor liposomes. ( a ) Inhibition of ATP-dependent [ 3 H] ATR transfer (10 μM) from ABCA4-containing donor proteoliposomes to acceptor liposomes with increasing concentrations of all- trans retinol or N -retinyl-PE. Donor proteoliposomes were reconstituted with ABCA4 purified from bovine ROS membranes. Percent-relative retinal transfer plotted as a mean with error bars representing±s.d. for n =3. ( b ) ATP-dependent transfer of [ 3 H] ATR from ABCA4-containing proteoliposomes composed of only DOPC (PC) or DOPC containing 30% DOPE (PE). Sigmoidal curve for PE was generated and yielded a K 0.5 =6.7 μM±0.3 with a Hill coefficient of 2.1±0.2. Percent relative retinal transfer plotted as a mean with error bars representing±s.d. for n =3. ( c ) Effect of increasing DOPE on the ATP-dependent transfer of [ 3 H] ATR from DOPC/DOPE proteoliposomes reconstituted with either WT ABCA4 or ABCA4-MM mutant. Data was plotted as mean with error bars representing±s.e.m. for n =6. ( d ) Absorption spectra of purified ABCA4 with bound retinoid substrate. Spectrum at neutral pH (solid line) shows a maximum of 360 nm characteristic of non-protonated N -retinylidene-PE. Treatment with HCl resulted in an absorption maximum of 440 nm characteristic of protonated N -retinylidene-PE. Treatment with NaCNBH 3 resulted in a shift to 330 nm characteristic of N -retinyl-PE. ( e ) HPLC chromatograph of NaCNBH 3 reduced retinoid substrate in ABCA4 with y -axis in absorbance units (A.U.). Retention time and absorption spectrum (inset) of the predominant peak (*) showing a λ -max at 330 nm. Full size image The Schiff base of N -retinylidene-PE in PC/PE vesicles undergoes protonation with an apparent p K a of 6.9 ( Supplementary Fig. S4 ). To investigate whether the protonated or non-protonated form of N -retinylidene-PE binds to ABCA4, ATR and PE were added to ABCA4 immobilized on a Rim3F4-Sepharose immunoaffinity matrix. After removing excess ATR and PE, ABCA4 with its bound substrate was released from the matrix with the 3F4-competing peptide for analysis by absorption spectroscopy. As shown in Fig. 3d , the bound retinoid substrate had an absorption maximum at 360 nm, characteristic of non-protonated N -retinylidene-PE. Treatment with HCl or NaCNBH 3 resulted in a shift in the absorption maximum to 440 or 330 nm, respectively, characteristic of protonated N -retinylidene-PE and N -retinyl-PE. Solvent extraction of NaCNBH 3 -treated ABCA4 followed by high-performance liquid chromatography (HPLC) chromatography confirmed that the reduced Schiff base compound was N -retinyl-PE ( Fig. 3e ). The transport activity of ABCA4 was also dependent on pH reaching a maximum at pH 8.0 ( Supplementary Fig. S5 ). Collectively, these studies indicate that the non-protonated form of N -retinylidene-PE is the retinoid substrate transported by ABCA4. ABCA4-mediated substrate transport from ROS discs To determine if ABCA4-mediated ATR transfer can occur from a more physiological system, we replaced the reconstituted proteoliposomes with closed ROS disc membrane vesicles ( Fig. 4a ), which retain their orientation with the cytoplasmic surface exposed to the buffer [18] , [31] , [32] . In this assay, disc vesicles comprised the dense fraction and acceptor lysosomes prepared in the absence of sucrose made up the light fraction. [ 3 H]-ATR rapidly partitioned between the disc and acceptor vesicles ( Fig. 4b ). Addition of ATP, but not AMP–PNP, resulted in a linear transfer of [ 3 H]-ATR to the acceptor vesicles. The rate of [ 3 H]-ATR transfer was dependent of ATR concentration yielding a sigmoidal curve with a K 0.5 of 6.8±0.3 μM, a V max of 4.9±0.1 nmol min −1 per mg protein, and a Hill coefficient of 1.8±0.1 ( Fig. 4c ). Importantly, the direction of transport was consistent with the movement of N -retinylidene-PE from the inner lumen leaflet to the outer cytoplasmic leaflet of the disc vesicles. 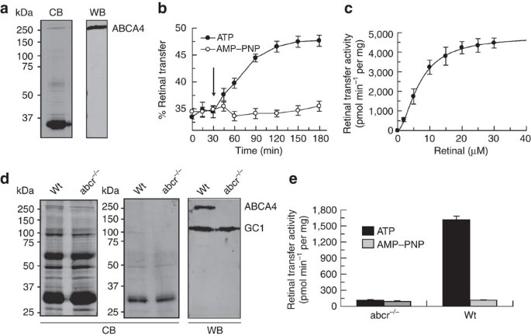Figure 4: ATP-dependent transfer of ATR from ROS discs to acceptor vesicles. (a) Coomassie blue stained SDS gel (CB) and western blot (WB) of bovine ROS disc vesicles used in the ATR transfer reactions. (b) Time course for the transfer of [3H] ATR from donor disc vesicles to acceptor vesicles. At 30 min, 5 mM ATP or AMP–PNP (arrow) was added to start the transfer reaction. A higher ATP concentration was required to compensate for the presence of non-specific ATPase in the disc membranes. Data plotted as a mean with error bars representing±s.d. forn=3. (c) ATP-dependent rate of [3H] ATR transfer (retinal transfer activity) from disc vesicles to acceptor liposomes as a function of ATR concentration. The best-fit sigmoidal curve was generated for aK0.5of 6.8±0.3 μM and aVmaxof 4.9±0.1 nmol min−1per mg protein, and yielded a Hill coefficient of 1.8±0.1. Data plotted as a mean with error bars representing±s.d. forn=3. (d) Coomassie blue (CB)-stained gels of ROS (left panel) and hypotonically lysed and washed discs (middle panel) from wild-type (Wt) andabca4knockout (abca4−/−) mice. Western blot (right panel) labelled for ABCA4 and guanylate cyclase 1 (GC1). ROS and disc membranes from WT andabca4−/−mice display similar protein profiles except for the absence of ABCA4 in theabca4−/−preparations as revealed by western blotting. (e) ATP-dependent [3H] ATR transfer from disc membranes of WT andabca4−/−mice to acceptor vesicles. Data plotted as a mean with error bars representing±s.e.m. forn=9. Figure 4: ATP-dependent transfer of ATR from ROS discs to acceptor vesicles. ( a ) Coomassie blue stained SDS gel (CB) and western blot (WB) of bovine ROS disc vesicles used in the ATR transfer reactions. ( b ) Time course for the transfer of [ 3 H] ATR from donor disc vesicles to acceptor vesicles. At 30 min, 5 mM ATP or AMP–PNP (arrow) was added to start the transfer reaction. A higher ATP concentration was required to compensate for the presence of non-specific ATPase in the disc membranes. Data plotted as a mean with error bars representing±s.d. for n =3. ( c ) ATP-dependent rate of [ 3 H] ATR transfer (retinal transfer activity) from disc vesicles to acceptor liposomes as a function of ATR concentration. The best-fit sigmoidal curve was generated for a K 0.5 of 6.8±0.3 μM and a V max of 4.9±0.1 nmol min −1 per mg protein, and yielded a Hill coefficient of 1.8±0.1. Data plotted as a mean with error bars representing±s.d. for n =3. ( d ) Coomassie blue (CB)-stained gels of ROS (left panel) and hypotonically lysed and washed discs (middle panel) from wild-type (Wt) and abca4 knockout (abca4 −/− ) mice. Western blot (right panel) labelled for ABCA4 and guanylate cyclase 1 (GC1). ROS and disc membranes from WT and abca4 −/− mice display similar protein profiles except for the absence of ABCA4 in the abca4 −/− preparations as revealed by western blotting. ( e ) ATP-dependent [ 3 H] ATR transfer from disc membranes of WT and abca4 −/− mice to acceptor vesicles. Data plotted as a mean with error bars representing±s.e.m. for n =9. Full size image To confirm that that the ATP-dependent transfer of ATR is mediated by ABCA4, we compared the ATR transfer reaction from disc membrane vesicles of WT mice with those of abca4 knockout mice. With the exception of ABCA4, the disc protein compositions were similar ( Fig. 4d ). ATP-dependent transfer of [ 3 H]-ATR was observed from WT disc membranes but not abca4 knockout membranes ( Fig. 4e ). ABCA4 functions as a PE importer ABCA4 reconstituted into PE-containing lipid vesicles exhibits basal ATPase activity in the absence of retinal [22] , [23] . We reasoned that this activity may be associated with the transport of a phospholipid across the lipid bilayer, a function which has been reported for other ABC transporters notably ABCB1 (P-glycoprotein) [33] . To test this, we used the well-established fluorescence spectroscopic technique to measure the active transport of 7-nitro-2-1,3-benzoxadiazol-4-yl-labelled (NBD-labelled) phospholipids across the lipid bilayer [33] , [34] , [35] , [36] . In this assay, ATP or its non-hydrolyzable analogue AMP–PNP was added to ABCA4 proteoliposomes containing NBD-labelled-PE, NBD-labelled-PC or NBD-labelled-PS. After 1 h, the impermeable reducing agent dithionite was added to selectively bleach NBD-labelled lipids on the outer leaflet. Complete bleaching of the NBD-labelled lipids was achieved by the addition of Triton X-100 ( Supplementary Fig. S6 ). The amount of NBD-labelled lipid transported to the outer leaflet was determined from the difference in fluorescence after dithionite addition between samples treated with ATP and AMP–PNP and expressed as a percentage of NBD-labelled lipid transported. When ABCA4 was reconstituted into PC vesicles containing NBD-labelled phospholipids, ATP-dependent transport was observed for NBD-labelled-PE, but not NBD-labelled-PS or NBD-labelled-PC ( Fig. 5a ). The direction of transport was from the lumen to the cytoplasmic leaflet of the vesicles similar to the direction of N -retinylidene-PE transport. NBD-labelled-PE transport increased with increasing NBD-labelled-PE incorporated into the proteoliposomes ( Fig. 5b ) and was suppressed by the addition of 30% unlabelled PE ( Fig. 5a ). Transport activity was not observed for the ATPase-defective mutant, ABCA4-MM. As in the case of N -retinylidene-PE transport, GTP could partially substitute for ATP and beryllium fluoride and NEM acted as strong inhibitors ( Fig. 5c ). 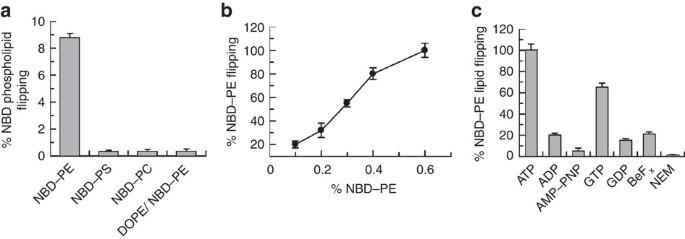Figure 5: PE flippase activity of ABCA4. (a) ABCA4 was reconstituted into DOPC vesicles containing 0.6% NBD-labelled-PE (NBD–PE), NBD-labelled-PS (NBD–PS), NBD-labelled-PC (NBD–PC) or 0.6% NBD-labelled-PE plus 30% unlabelled DOPE (DOPE/NBD–PE). Data plotted as a mean with error bars representing±s.e.m.,n=9 for three independent experiments. (b) Dependence of NBD-labelled-PE flipping or transport across the bilayer as a function of % NBD-labelled-PE. Percent-relative PE flipping plotted as a mean with error bars representing±s.d. forn=3. (c) The effect of nucleotides (1 mM), beryllium fluoride (BeFx0.2 mM) and NEM (10 mM) on the NBD-labelled-PE flippase activity. Percent-relative NBD-PE flipping plotted as a mean with error bars representing±s.d. forn=3. Figure 5: PE flippase activity of ABCA4. ( a ) ABCA4 was reconstituted into DOPC vesicles containing 0.6% NBD-labelled-PE (NBD–PE), NBD-labelled-PS (NBD–PS), NBD-labelled-PC (NBD–PC) or 0.6% NBD-labelled-PE plus 30% unlabelled DOPE (DOPE/NBD–PE). Data plotted as a mean with error bars representing±s.e.m., n =9 for three independent experiments. ( b ) Dependence of NBD-labelled-PE flipping or transport across the bilayer as a function of % NBD-labelled-PE. Percent-relative PE flipping plotted as a mean with error bars representing±s.d. for n =3. ( c ) The effect of nucleotides (1 mM), beryllium fluoride (BeF x 0.2 mM) and NEM (10 mM) on the NBD-labelled-PE flippase activity. Percent-relative NBD-PE flipping plotted as a mean with error bars representing±s.d. for n =3. Full size image Stargardt mutations decrease transport activity To gain further insight into the molecular mechanisms underlying ABCA4-mediated transport activity and Stargardt disease, we examined the functional properties of ABCA4-containing G863A and N965S mutations associated with Stargardt disease and Walker A mutations, K969M in NBD1, K1978M in NBD2 and the double mutant K969M/1978M. The K1978M mutant expressed at the same level as WT ABCA4, whereas the G863A, N965S, K969M and K969M/K1978M mutants expressed within 50% that of WT ABCA4. All mutants could be readily purified by immunoaffinity chromatography ( Fig. 6a ). 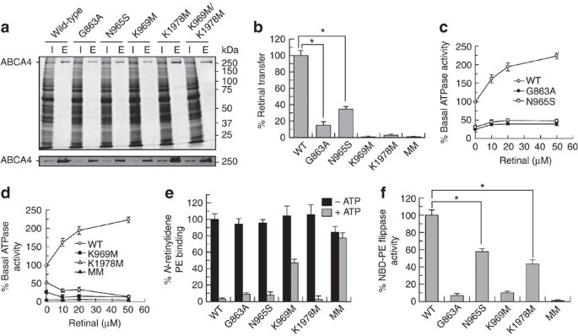Figure 6: Effect of Walker A and Stargardt mutations on ATR transfer activity. (a) Wild-type and mutant ABCA4 containing a 1D4 epitope were expressed in HEK293T cells and purified on a Rho-1D4 immunoaffinity matrix. Commassie blue stained gel (upper) and western blot (lower) for the various ABCA4 mutants. Lanes labelled I (input) are the HEK293T detergent solubilized extract applied to the immunoaffinity matrix. Lanes labelled E (eluted) are fractions released from the immunoaffinity matrix with the 1D4 peptide. (b) ATP-dependent [3H] ATR transfer activity for the various mutants relative to wild-type ABCA4. Percent-relative retinal transfer plotted as a mean with error bars representing±s.e.m. forn=9 from three independent experiments. Statistically significant differences (P<0.05) are denoted with * for the indicated data sets as determined by analysis of variance (ANOVA). (c) ATPase activity of the Stargardt mutants as a function of ATR concentration and expressed as a % of WT activity in the absence of retinal. Data plotted as a mean with error bars representing ± s.e.m. forn=6 from two independent experiments. (d) ATPase activity of the Walker A mutants as a function of ATR concentration. Data plotted as a mean with error bars representing±s.e.m. forn=6 from two independent experiments. (e) Binding ofN-retinylidene-PE to immobilized WT and mutant ABCA4 and release by 0.5 mM ATP. Binding normalized to WT ABCA4. Data plotted as a mean±s.e.m. forn=9 from three independent experiments. (f) ATP-dependent flippase activity of NBD-labelled-PE by mutant ABCA4. Percent-relative PE flipping plotted as a mean with error bars representing±s.e.m. forn=9 from three independent experiments. Statistically significant differences (P<0.05) are denoted with * as determined for the indicated data sets by ANOVA. Figure 6: Effect of Walker A and Stargardt mutations on ATR transfer activity. ( a ) Wild-type and mutant ABCA4 containing a 1D4 epitope were expressed in HEK293T cells and purified on a Rho-1D4 immunoaffinity matrix. Commassie blue stained gel (upper) and western blot (lower) for the various ABCA4 mutants. Lanes labelled I (input) are the HEK293T detergent solubilized extract applied to the immunoaffinity matrix. Lanes labelled E (eluted) are fractions released from the immunoaffinity matrix with the 1D4 peptide. ( b ) ATP-dependent [ 3 H] ATR transfer activity for the various mutants relative to wild-type ABCA4. Percent-relative retinal transfer plotted as a mean with error bars representing±s.e.m. for n =9 from three independent experiments. Statistically significant differences ( P <0.05) are denoted with * for the indicated data sets as determined by analysis of variance (ANOVA). ( c ) ATPase activity of the Stargardt mutants as a function of ATR concentration and expressed as a % of WT activity in the absence of retinal. Data plotted as a mean with error bars representing ± s.e.m. for n =6 from two independent experiments. ( d ) ATPase activity of the Walker A mutants as a function of ATR concentration. Data plotted as a mean with error bars representing±s.e.m. for n =6 from two independent experiments. ( e ) Binding of N -retinylidene-PE to immobilized WT and mutant ABCA4 and release by 0.5 mM ATP. Binding normalized to WT ABCA4. Data plotted as a mean±s.e.m. for n =9 from three independent experiments. ( f ) ATP-dependent flippase activity of NBD-labelled-PE by mutant ABCA4. Percent-relative PE flipping plotted as a mean with error bars representing±s.e.m. for n =9 from three independent experiments. Statistically significant differences ( P <0.05) are denoted with * as determined for the indicated data sets by ANOVA. Full size image All mutants reconstituted into proteoliposomes showed a severe loss in N -retinylidene-PE transfer activity with the three Walker A mutants showing essentially undetectable activity and the G863A and N965S Stargardt mutants displaying ~18 and 37% of WT activity ( Fig. 6b ). Retinal-stimulated ATPase activities of these mutants were also analysed ( Fig. 6c,d ) with Stargardt mutants showing very modest retinal stimulation and Walker A mutants showing some inhibition of ATPase activity with increasing retinal concentration. Next we studied the effect of the mutations on N -retinylidene-PE binding to immobilized ABCA4 and its release by ATP ( Fig. 6e ). All mutants bound N -retinylidene-PE at similar levels to WT ABCA4. Addition of ATP resulted in release of the substrate from the G863A, N965S and K1978M mutants, but impaired release from the K969M mutant and no significant release from the K969M/K1978M double mutant. Finally, we determined the effect of these mutations on NBD-labelled-PE flippase activity. All mutants showed significantly reduced PE flippase activity in general agreement with their loss in basal ATPase activity ( Fig. 6f ). In this study, we provide direct biochemical evidence for the full eukaryotic ABC transporter ABCA4 functioning as an 'importer' translocating its substrates N -retinylidene-PE and PE from the lumen to the cytoplasmic side of photoreceptor disc membranes. This is supported in three different experimental systems. First, the addition of ATP, but not AMP–PNP, to the outside of donor vesicles reconstituted with purified ABCA4 promotes the time-dependent transfer of retinal (ATR) to acceptor liposomes. As ATP is negatively charged, it can only interact with the NBDs of ABCA4 exposed on the outside of the vesicle, an orientation equivalent to the cytoplasmic side of biological membranes, and drive transfer of retinal to acceptor liposomes, a direction expected for an importer. The reaction is specific for functional ABCA4, as ATP-dependent retinal transfer activity is not observed for ATPase-defective ABCA4 mutants [37] . Furthermore, NEM and beryllium fluoride both of which inhibit the ATPase activity of ABCA4 [38] also abolish ABCA4-mediated retinal transfer activity. Second, ATP-dependent retinal transfer is observed from bovine and WT mouse photoreceptor disc membranes, but not abca4 knockout disc membranes. Third, ABCA4 reconstituted into lipid vesicles can actively flip PE from the inner to the outer surface of vesicles, a direction that is consistent with an 'import' direction of PE transport. All mammalian and mostly all well-characterized eukaryotic ABC transporters have been shown to act as 'exporters' extruding or flipping their substrates from the cytoplasmic to the extracellular or lumen side of biological membranes [33] , [36] , [39] , [40] , [41] , [42] . Exceptions are found in the plant kingdom where several ABC transporters have been reported to function as importers [2] , [43] . Direct substrate transport has not been measured for other members of the ABCA subfamily, but cell-based studies have suggested that these transporters function as lipid exporters [44] , [45] , [46] . In particular ABCA1, which is 50% identical in sequence to ABCA4, is known to facilitate the export of cholesterol and phospholipids from cells to Apo-A1 although this remains to be confirmed at a biochemical level. Indeed, if all other ABCA transporters are found to function as lipid exporters, it will be of interest to determine the molecular basis, which defines ABCA4 as a unique importer in this subfamily. Although the assay developed in this study measures the transfer of retinal from donor to acceptor vesicles, the true substrate for ABCA4 is N -retinylidene-PE. Retinal is a hydrophobic compound, which readily diffuses across the lipid bilayer and hence does not need a specific transporter. However, retinal readily reacts with PE, which comprises about 40% of the phospholipid in disc membranes to form N -retinylidene-PE, a compound which cannot diffuse across membranes. We have confirmed earlier studies that ABCA4 tightly binds N -retinylidene-PE in the absence of ATP [26] , and further show here that it binds the non-protonated form of N -retinylidene-PE on the basis of spectral measurements and HPLC analysis. Furthermore, N -retinyl-PE, the stabilized covalent analogue of N -retinylidene-PE, competes with N -retinylidene-PE for binding to ABCA4 [24] , and inhibits its transport activity. Collectively, our studies suggest that the addition of retinal to a mixture of PE-containing donor and acceptor vesicles results in its rapid partitioning between these vesicle populations with retinal and PE in dynamic equilibrium with N -retinylidene-PE. ABCA4 catalyses the active transport of N -retinylidene-PE from the inside to the outside of donor proteoliposomes or disc vesicles as a rate-limiting step. The increase in N -retinylidene-PE on the outer leaflet of the donor proteoliposomes coupled with its dissociation into retinal and PE leads to the observed ATP-dependent transfer of retinal to acceptor liposomes. A number of high-resolution structures of prokaryotic and eukaryotic ABC transporters, both importers and exporters, have been determined by X-ray crystallization, some bound with ATP or their transport substrate [47] , [48] , [49] , [50] . These studies have led to the proposal that both types of transporters use broadly similar alternating access transport mechanisms [5] , [6] . In the absence of ATP, exporters bind their substrate at a high-affinity-binding site accessible to the cytoplasmic side of the membrane. The binding of ATP results in the dimerization of the NBDs, a process that is coupled to a conformational change in the transmembrane domains and conversion to low-affinity outwardly oriented binding site and dissociation of the substrate from the transporter on the exocytoplasmic side of the membrane. ATP hydrolysis together with the release of ADP and P i results in another conformational change, which resets the protein to its initial state. Prokaryotic importers, on the other hand, typically bind their substrate on the exocytoplasmic side of the membrane in the presence of ATP, often facilitated through interaction with a substrate-binding protein. Hydrolysis of ATP leads to the conversion to a low-affinity inward-oriented-binding site and release of the substrate on the cytoplasmic side of the membrane. Our studies suggest a model in which ABCA4 in the absence of ATP and a substrate-binding protein has a high-affinity outward (lumen)-facing site for the binding of N -retinylidene-PE or PE [24] . The binding of ATP induces a protein conformational change, which switches the high-affinity site to a low-affinity inward (cytoplasmic)-facing site enabling N -retinylidene-PE or PE to be released on the cytoplasmic leaflet of the disc membrane. In this model, ATP hydrolysis would restore the initial conformation of ABCA4 to initiate another cycle of transport. This model is supported by our studies on the effect on Stargardt mutations on the properties of ABCA4. The binding of N -retinylidene-PE and its release by ATP is not affected by the G863A and N965S mutations ( Fig. 6e ), but the basal- and retinal-stimulated ATPase activity and ATP-dependent retinal transfer activity are significantly reduced. Similarly, mutations in the Walker A motif also abolish retinal-stimulated ATPase activity and ATP-dependent retinal transfer activity without affecting N -retinylidene-PE binding and with the exception of the double mutant not drastically affecting substrate release by ATP. Previous in vitro biochemical studies have relied on the purification and reconstitution of ABCA4 into liposomes for analysis of its basal- and retinal-stimulated ATPase activities. Such activities could not be accurately measured in disc membrane preparations due to the high non-specific ATPase activity in these preparations [34] . However, as shown in this study active retinoid transport activity of ABCA4 can be measured in disc membranes resulting in a V max of 4.9 nmol min −1 per mg protein. As ABCA4 represents about 5% of the disc membrane protein by weight [21] , this suggests the specific activity of ABCA4 is about 98 nmol min −1 per mg, a value comparable to the value of ~53 nmol min −1 per mg for ABCA4 derived from kinetic measurements of proteoliposomes having 75% of the ABCA4 oriented with its NBDs accessible to ATP ( Supplementary Fig. S7 ). The turnover numbers for the reduction of all- trans retinal to all- trans retinol by the retinol dehydrogenase Rdh8 have been reported to range from 0.3 min −1 ( in vitro ), 0.06 min −1 ( in situ ) and 0.0003 min −1 ( in vitro ) [51] , [52] , [53] . The estimated turnover number (24.5 min −1 ) for ABCA4 in disc membranes is several orders of magnitude higher. Given that ABCA4 and Rdh8 occur at 1:120 and 1:140 of rhodopsin levels [21] , [54] , this suggests that N -retinylidene-PE transfer is at least two orders of magnitude faster than the reduction reaction. On this basis, ABCA4 appears to assure that all of the ATR is made accessible on the cytoplasmic side of disc membranes where it can be either reduced to retinol by Rdh8 or diffuse from the disc and undergo reduction by retinol dehydrogenase isoforms localized in different photoreceptor subcellular compartments ( Fig. 7 ). Interestingly, the dependence of N -retinylidiene-PE transport activity on retinal concentration results in a sigmoidal curve ( Figs 2b and 3b ), suggesting that retinal can act as an allosteric activator of retinoid transport. This is consistent with earlier studies showing that ABCA4 contains a binding site for retinal, which is distinct from the N -retinylidene-PE-binding site [24] , [55] . 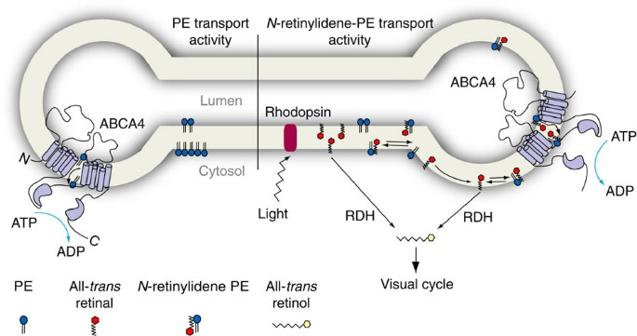Figure 7: Schematic diagram showing ABCA4 functioning in the transport ofN-retinylidene-PE and PE across the ROS disc membrane. Left: ABCA4 shown to function in the transport of PE from the lumen to the cytoplasmic leaflet of the disc membrane. Right: ABCA4 shown to function in the transport ofN-retinylidene-PE from the lumen to the cytoplasmic side of the disc membrane following the photobleaching of rhodopsin.N-retinylidene-PE dissociates into ATR and PE on the cytoplasmic side of the disc membrane with ATR subsequently being reduced to retinol by the retinol dehydrogenase (RDH) before entering the visual cycle for regeneration of 11-cisretinal. Figure 7: Schematic diagram showing ABCA4 functioning in the transport of N -retinylidene-PE and PE across the ROS disc membrane. Left: ABCA4 shown to function in the transport of PE from the lumen to the cytoplasmic leaflet of the disc membrane. Right: ABCA4 shown to function in the transport of N -retinylidene-PE from the lumen to the cytoplasmic side of the disc membrane following the photobleaching of rhodopsin. N -retinylidene-PE dissociates into ATR and PE on the cytoplasmic side of the disc membrane with ATR subsequently being reduced to retinol by the retinol dehydrogenase (RDH) before entering the visual cycle for regeneration of 11- cis retinal. Full size image In addition to flipping N -retinylidene-PE, ABCA4 can also flip PE across membranes in the same 'import' direction ( Fig. 7 ), an activity that is related to the basal ATPase activity of ABCA4 [22] , [23] . The distribution of phospholipids across the disc membrane is not clearly resolved. Several earlier studies have reported an asymmetrical distribution of PS and PE with 67–87% of the PE and 77–88% of PS on the cytoplasmic leaflet [56] , [57] . Other studies suggest a more symmetrical distribution of PE and a modest asymmetry for PS possibly arising from ATP-independent flippase activity of opsin [58] , [59] . In the former case, ABCA4 may contribute to the generation and maintenance of PE asymmetry, whereas in the latter case, this activity may be overwhelmed by the flippase activity of opsin. More studies are needed to resolve phospholipid asymmetry in photoreceptor membranes and the involvement of ABCA4 in this process. Purification of ABCA4 The Rim3F4 monoclonal antibody conjugated to Sepharose 2B was used to isolate ABCA4 from 3-[(3-cholamidopropyl)dimethylammonio]-2-hydroxy-1-propanesulfonate (CHAPS)-solubilized bovine ROS membranes and the Rho1D4 monoclonal antibody conjugated to Sepharose 2B was used to purify WT and mutant ABCA4 containing a C-terminal 9-amino-acid 1D4 tag (T-E-T-S-Q-V-A-P-A) from CHAPS-solubilized, transfected HEK293T as described previously [22] , [30] . In each case, the purified ABCA4 was directly used for reconstitution into proteoliposomes. Preparation of proteoliposomes and acceptor liposomes For proteoliposomes, dioleoylphosphatidylcholine (DOPC), dioleoylphosphatidylethanolamine (DOPE) and porcine brain polar lipid (BPL) obtained from Avanti Polar Lipids were mixed at a weight ratio of 6:2:2 and dried under N 2 . BPL was used in our studies, as earlier studies suggested that this phospholipid mixture having variable fatty acyl groups was required to stabilize functional ATPase activity of ABCA4 [23] . The donor lipids were resuspended at a concentration of 5 mg ml −1 in buffer containing 20 mM 4-(2-hydroxyethyl)-1-piperazineethanesulfonic acid (HEPES) buffer, pH 8.0, 150 mM NaCl, 2 mM MgCl 2 and 18 mM CHAPS with bath sonication. The donor lipids and the ABCA4 protein (in CHAPS detergent with dithiothreitol (DTT)) were mixed to yield a final protein-to-lipid ratio of 1:100 (wt/wt) with a reduction in CHAPS concentration to 6 mM. After incubation at 4 °C for 1 h, the detergent was removed by dialysis at 4 °C over a 24-h period with a minimum of three changes of buffer containing 10 mM HEPES, pH 8.0, 150 mM NaCl, 2 mM MgCl 2 and 1 mM DTT. For acceptor liposomes, DOPC and DOPE at a weight ratio of 7:3 were resuspended in 20 mM HEPES pH 8.0, 150 mM NaCl, 2 mM MgCl 2 and 18 mM CHAPS with 300 mM sucrose, incubated at room temperature for 4 h, and dialysed as above against 10 mM HEPES, pH 8.0, 300 mM sucrose, 2 mM MgCl 2 and 1 mM DTT. Vesicle sizes were measured on a Nicomp Submicron Particle Sizer Model 370. Proteoliposomes displayed a narrow Gaussian distribution with vesicles having a mean diameter of 74±18.8 nm; liposomes containing 10% sucrose showed a wider distribution in the range of 50–450 nm and a mean diameter of 203.2±115.8 nm. ATP-dependent retinoid transfer between liposomes [ 3 H] all- trans retinal ([ 3 H]-ATR) or [ 3 H] all- trans retinol (1.68 kBq, 3.36 GBq mmol −1 ) was dried under N 2 for 5 min, and subsequently incubated with donor proteoliposomes for 2 h at 4 °C. Reconstituted proteoliposomes (~40 μl) containing approximately 1 μg of protein were added to 200 μl of buffer B (20 mM HEPES, pH 8.0, 150 mM NaCl, 3 mM MgCl 2 and 1 mM DTT). Before the reaction, a total of 200 μg, ~20 μl, of acceptor liposomes were added to the reaction mixture reducing the external sucrose concentration to 30 mM. The tubes were wrapped in tin-foil and reaction was typically carried out for 60 min at 37 °C in the presence of 1 mM ATP or AMP–PNP. The reaction mixture was then added to the top of a centrifuge tube containing 2.5 ml separation buffer (20 mM HEPES, pH 8.0, 75 mM NaCl, 150 mM sucrose) and centrifuged using a Beckman TLA110.4 rotor at 100,000 g for 20 min. The difference in the densities of the two vesicles was sufficient for separation by centrifugation. The supernatant was transferred to a scintillation vial and the pellet was resuspended in 200 μl of buffer B and transferred to a second scintillation vial. The radioactivity of the fractions was determined by liquid scintillation counting. ABCA4 proteoliposomes with acceptor vesicles in the absence of nucleotide was used as a control to subtract the background counts primarily arising from the spontaneous [ 3 H]-retinoid partitioning between the proteoliposomes and liposomes from nucleotide-treated reactions. For substrate competition assays, ATR was used at 10 μM together with increasing concentrations of unlabelled all- trans retinol and N -retinyl PE. Preparation of ROS disc vesicles Bovine ROS (25 mg) purified from previously frozen retina [24] were used to prepare disc vesicles by the Ficoll centrifugation procedure [31] . The sealed disc vesicles collected at the Ficoll–water interface were washed with 20 mM Tris, pH 7.6 and stored in 20 mM Tris, pH 7.6, containing 600 mM sucrose. Mouse retina dissected from 3-month-old wild-type and abca4 knockout ( abca4 −/− ) mice [60] and resuspended in 10 mM Tris, pH 7.6, 20% sucrose. For each experiment, five retinas from WT and abca4 −/− were resuspended in 0.25 ml buffer was vortexed for 30–60 s. The samples were then centrifuged at 200 g for 40 s, and the supernatant containing ROS was gently removed. This was repeated six times. The supernatant was loaded on 50% sucrose in 20 mM Tris, pH 7.6 and centrifuged in a TLA55 rotor at 40,000 g for 45 min at 4 °C. ROS were collected on top of the 50% sucrose buffer layer, washed three times in buffer (10 mM HEPES pH 8.0, 100 mM NaCl, 1 mM MgCl 2 ) and layered on 20 mM Tris, pH 7.6, 30% sucrose for a second round of purification. The ROS was subjected to osmotic lysis treatments in 10 mM Tris, pH 7.6, 1 mM EDTA for 1 h and in 2 mM Tris, pH 7.6 for 5 h. The ROS disc vesicles were washed three times by centrifugation at 40,000 g in a TLA110 rotor and treated with neutralized 3 mM hydroxylamine for 10 min. The disc vesicles were subsequently washed three times to remove excess hydroxylamine and retinaloxime and resuspended in buffer C (10 mM HEPES pH 8.0, 100 mM NaCl, 300 mM sucrose, 1 mM MgCl 2 ) for the retinal transfer assays. Retinoid transfer from disc vesicles to acceptor liposomes For retinoid transfer studies from ROS disc vesicles, acceptor liposomes consisting of DOPC/DOPE (7:3) were prepared by sonication in buffer B. Bovine vesicles were bleached and the endogenous retinal was derivatized with 5 mM of freshly neutralized hydroxylamine for 30 min at 25 °C. The bovine vesicles were then washed thrice with buffer C at 50,000 g and resuspended in the same buffer. [ 3 H]-ATR (1.68 kBq, 3.36 GBq mmol −1 ) was dried under N 2 for 5 min and incubated together with unlabelled ATR (2.5–30 μM) with 30 μg of bovine ROS disc vesicles for 1 h at 30 °C with 200 μg acceptor vesicles, 1 mM ouabain, 5 mM ATP or AMP–PNP or buffer (control). A higher concentration of nucleotide was used in these studies to compensate for the ouabain-insensitive endogenous ATPase activity of ROS disc membranes. Reactions were then layered on top of 2.5 ml of separation buffer containing 10 mM HEPES, pH 8.0, 600 mM sucrose and centrifuged at 100,000 g for 20 min. After the separation, the supernatant was removed and the pelleted ROS disc vesicles were resuspended in buffer C and radioactivity determined with liquid scintillation counting. In this case, the ROS disc vesicles were present in the pellet, whereas the acceptor vesicles remained in the supernatant atop the sucrose gradient. Control reactions with acceptor vesicles and ROS vesicles (bovine/mice) and no nucleotide addition were used as control to subtract radioactivity from retinal partitioning between vesicle populations. At least three independent experiments were performed for each transfer reaction. NBD-labelled phospholipid translocation assay Samples were prepared by adding 40 μl proteoliposomes with 0.6% NBD-labelled lipid (w/w) to 50 μl of buffer containing 20 mM HEPES, pH 7.0, 100 mM NaCl, 5 mM MgCl 2 , 1 mM DTT. To initiate transport, ATP (1 mM) or AMP–PNP (1 mM) was added to the proteoliposomes for 1 h at 37 °C. The fluorescence was recorded with a Varian spectrofluorometer using excitation and emission wavelengths of 468 and 540 nm, respectively. After a baseline was established, 4 mM of sodium dithionite solution in 1 M Tris–HCl (pH 10.0) was added to quench the fluorescence of NBD-labelled lipids in the outer leaflet of the proteoliposomes. When a baseline was re-established, the proteoliposomes were permeabilized by adding 1% Triton X-100 (TX-100). The net percent NBD-labelled lipid translocated in the proteoliposomes was calculated from the difference that was accessible to dithionite (outer leaflet), or protected from dithionite (inner leaflet), using the following equations. where F T is the total fluorescence of the sample before addition of dithionite, F D is the fluorescence of the sample following quenching with dithionite and F 0 is any residual fluorescence of the sample following permeabilization with TX-100. How to cite this article: Quazi, F. et al . ABCA4 is an N -retinylidene-phosphatidylethanolamine and phosphatidylethanolamine importer. Nat. Commun. 3:925 doi: 10.1038/ncomms1927 (2012).